Targeted inhibition of fascin function blocks tumour invasion and metastatic colonization One of the key steps during tumour metastasis is tumour cell migration and invasion, which require actin cytoskeletal reorganization. Among the critical actin cytoskeletal protrusion structures are the filopodia, which act like cell sensory organs to communicate with the extracellular microenvironment and participate in fundamental cell functions such as cell adhesion, spreading and migration in the three-dimensional environment. Fascin is the main actin-bundling protein in filopodia. Using high-throughput screening, here we identify and characterize small molecules that inhibit the actin-bundling activity of fascin. Focusing on one such inhibitor, we demonstrate that it specifically blocks filopodial formation, tumour cell migration and invasion in vitro , and metastasis in vivo . Hence, target-specific anti-fascin agents have a therapeutic potential for cancer treatment. In recent years, significant progress has been made in the treatment of cancer, particularly with the development of targeted therapy. However, there is very little advancement in the area of blocking tumour metastasis, which remains the primary cause of mortality of cancer patients [1] , [2] . Metastasis is comprised of a series of events that a primary tumour spreads from its initial site to secondary tissues/organs [3] . This invasion-metastasis cascade includes cell migration/invasion, intravasation, survival in the circulation, arrest in a distant capillary bed and extravasation into and colonization within the organ parenchyma. Inhibition of any one of these steps could block the entire metastatic process. Tumour cell migration and invasion are critical steps in metastasis [4] , [5] , [6] , [7] , [8] , [9] , [10] . Migration provides tumour cells the ability to leave the primary tumour bed (local invasion), enter into blood vessels, then exit the circulation and infiltrate the distant tissues/organs. For cell migration and invasion to proceed, actin cytoskeleton must be reorganized by forming actin polymers and bundles to dynamically change cell shapes [11] . Individual actin filaments are flexible and insufficient for membrane protrusion. Bundling of actin filaments provides rigidity against the compressive force from the plasma membrane [12] . One of the main actin filament-based membrane protrusions is filopodia [13] . Filopodia are finger-like plasma membrane protrusions that are formed upon remodelling of the actin cytoskeleton beneath the plasma membrane [13] . They can be viewed as a sensory organ of the cells that are used to detect and assimilate signals as well as to explore and move into the surrounding microenvironment [14] , [15] , [16] . Filopodia are also involved in transporting signalling proteins within tissues over a long range [16] . Metastatic tumour cells are rich in filopodia, and the number of which correlates with their invasiveness [17] , [18] . Recently, filopodium-like protrusions have also been implicated to be critical for metastatic tumour cells to colonize in the secondary tissues or organs [19] . Fascin is the primary actin cross-linker in filopodia and has no amino-acid sequence homology with other actin-binding proteins [20] , [21] , [22] , [23] , [24] , [25] . It has a molecular mass of ∼ 55 kDa, functions as a monomer and is required to maximally cross-link the actin filaments into straight, compact and rigid bundles, to impart distinct mechanical stiffness to actin bundles [26] , [27] . Fascin holds 10–30 parallel actin filaments together to form filopodia 60–200 nm in diameter [13] . Elevated levels of fascin have been found in many types of metastatic tumours and are correlated with clinically aggressive phenotypes, poor prognosis and shorter survival [28] , [29] , [30] . Human fascin expression is low or absent in normal adult epithelial cells, but highly expressed in embryonic stages [31] , [32] . Fascin gene-knockout mice are normal, likely due to the functional compensation of other actin-bundling proteins during embryonic development [33] . Fascin point mutations in Drosophila (the singed mutants) cause defective actin bundling and lead to curled bristles, waved body hairs and impaired oogenesis [34] . Furthermore, when ectopically expressed, fascin promotes tumour cell migration, invasion and metastasis [28] . Moreover, it has been suggested that upregulation of fascin is part of the programme of epithelial-to-mesenchymal transition that confers motility and invasion properties on tumour cells [29] . Therefore, fascin has been suggested as a therapeutic target for blocking tumour cell migration, invasion and metastasis [31] , [32] , [35] , [36] , [37] , [38] , [39] , [40] , [41] , [42] , [43] . Previously, we solved the X-ray crystal structures of the wild-type fascin and four fascin mutants to define the active and inactive configurations of fascin, and revealed the structural basis for the conformational changes of fascin during the actin-binding process [35] , [44] . From a systematic mutagenesis study of 100 fascin mutants, we identified at least two major actin-binding sites on fascin, and that each of these actin-binding sites is essential for the filopodial formation in cells [44] . We used cryo-electron tomography and analysed the in vitro reconstituted unconstrained three-dimensional (3D) bundles formed by fascin and actin filaments. These bundles consisted of a hexagonal lattice of parallel actin filaments where fascin formed the cross-bridges, and these bundles were similar to the filopodial bundles isolated from native tissues/cells [44] . Here we screened chemical libraries and identified small-molecule compounds that specifically inhibit the biochemical function of fascin to bundle actin filaments. These inhibitors also impair the cellular function of fascin of inducing the formation of filopodia in two-dimensional and 3D environment. Furthermore, the small-molecule inhibitor blocks breast tumour cell migration, invasion and metastasis. Our data demonstrate that fascin inhibitors could be developed to inhibit metastatic dissemination. Identification of small-molecule inhibitors of fascin Previously, using protein affinity purification, we had identified fascin as a protein target of some migrastatin (a natural product) analogues, which inhibit tumour cell migration, invasion and metastasis [35] . Owing to the unexpected nature of potential toxicity of small-molecule drugs, it is the best and usual practice of drug development to have more than one class of chemical compounds for a given protein target. The migrastatin analogues that we have previously investigated belong to a class of chemical compounds with similar core chemical scaffold. Therefore, we screened chemical libraries to identify new compounds that inhibit the actin-bundling activity of fascin and are structurally different from migrastatin analogues. To identify small-molecule inhibitors of fascin for future clinical applications and for in vivo biological function studies of fascin, we have screened chemical libraries to identify compounds that inhibit the actin-bundling activity of fascin. Instead of identifying small-molecule compounds that bind to fascin, we have chosen to identify small molecules that inhibit the function of fascin to bundle actin. The rationales were: (i) It is the actin-bundling activity of fascin that is important for tumour cell migration and invasion. (ii) Based on the X-ray crystal structure of fascin, there are many potential binding sites on fascin for small molecules, in addition to the two main actin-binding pockets [44] . Some fascin-binding compounds might not inhibit the actin-bundling function of fascin. We developed an imaging-based assay where we could observe the fascin-mediated actin bundles ( Fig. 1 ). This method was an adaptation of a method that we used previously [35] , [44] . Because the F-actin filaments or F-actin bundles bear negative charges, we reasoned that a positively charged surface would be able to capture the F-actin filaments and bundles ( Fig. 1a,b ). By labelling F-actin with phalloidin-conjugated with fluorescent dye, we could visualize the F-actin structures using fluorescent microscopy ( Fig. 1b,c ). Actin bundles formed by fascin were long and thick in shape. In contrast, in the absence of fascin, actin filaments organized into a network of short and thin curved threads ( Fig. 1b ). We then titrated the concentrations of both F-actin and fascin, and found that fascin-mediated actin bundles were most distinct when the final concentrations of fascin and F-actin were close to 0.2 μM, with a molar ratio of 1:1. The assay displayed striking differences between images with and without fascin, showing its potential to be developed into a high-content imaging assay ( Fig. 1c,d ). 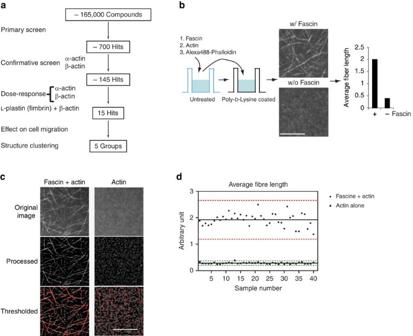Figure 1: Identification of small-molecule inhibitors of the actin-bundling function of fascin. (a) Summary of the screening strategy. (b) Outline of the HTS assay. (c) Examples of image acquisition and processing. Processed images were with homogenous illumination after shading correction and background subtraction. Thresholded images: A threshold of the grey values was applied, and parts of the images that have grey values between low and high limits were highlighted in red. (Details are in the Methods.) (d) Reproducibility of the HTS assay showing results from 40 different experiments (with or without fascin). The average fibre length of 40 samples in the presence (·) or absence (□) of fascin. The solid black horizontal lines show the means of the samples. Dotted red or green lines display 3 standard deviations (s.d.) from the mean of each data set (red for samples with fascin, and green for samples without fascin). Scale bars, 25 μm. Figure 1: Identification of small-molecule inhibitors of the actin-bundling function of fascin. ( a ) Summary of the screening strategy. ( b ) Outline of the HTS assay. ( c ) Examples of image acquisition and processing. Processed images were with homogenous illumination after shading correction and background subtraction. Thresholded images: A threshold of the grey values was applied, and parts of the images that have grey values between low and high limits were highlighted in red. (Details are in the Methods.) ( d ) Reproducibility of the HTS assay showing results from 40 different experiments (with or without fascin). The average fibre length of 40 samples in the presence (·) or absence (□) of fascin. The solid black horizontal lines show the means of the samples. Dotted red or green lines display 3 standard deviations (s.d.) from the mean of each data set (red for samples with fascin, and green for samples without fascin). Scale bars, 25 μm. Full size image During the screening, four images were taken for each well. The shading correction (processed) and background subtraction (thresholded) produced images with homogenous illumination ( Fig. 1c ). The microscopic actin-bundling assay was then optimized and miniaturized in a 384-well format for adaptation to high throughput screening (HTS). We carried out a large-scale primary screen of ∼ 165,000 compounds from the High-Throughput Screening Resource Center (Rockefeller University) at the compound concentration of 30 μM. A total of 753 compounds resulted in images looked like those of actin alone, indicating these compounds were most likely to specifically inhibit the actin-bundling activity of fascin; that was ∼ 0.5%, a reasonable hit rate in HTS ( Fig. 1a ). Individual hits were re-arrayed in 384-well plates with double sampling for each hit (two times with muscle α-actin proteins; two times with non-muscle β-actin proteins). Those (145 out of 753) giving a reproducible activity were used to produce 10-point dose–response curves ranging from 100 nM to 50 μM, with triplicate sampling (three times with α-actin proteins; three times with β-actin proteins). Active compounds of interest (15 out 145) for further study were defined as those with a reproducible IC 50 of less than 10 μM. In addition, a counter screen was carried out on those 15 compounds to evaluate their specificity against L-plastin, another actin-bundling protein. In this paper, we focused on one compound N-(1-(4-(trifluoromethyl)benzyl)-1H-indazol-3-yl)furan-2-carboxamide as an example due to its drug-like structure. We will refer to this compound as G2 here ( Fig. 2a ). The chemical structure of G2 was confirmed by NMR. G2 inhibited the actin-bundling activity of fascin (half-maximal inhibitory concentration (IC 50 ), 5 ∼ 8 μM), but not L-plastin (IC 50 >100 μM; Fig. 2b,d ). These data demonstrate that G2 inhibits the actin-bundling function of fascin, and has no inhibitory effect on actin polymerization itself and the actin-bundling activity of L-plastin. 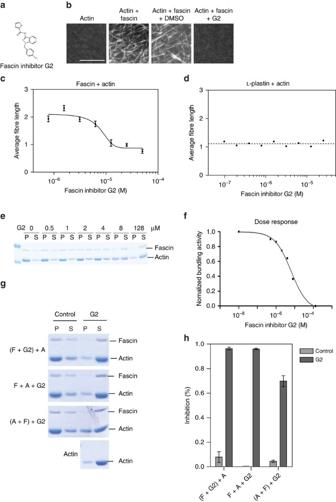Figure 2: Inhibition of the actin-bundling function of fascin by G2. (a) Chemical structure of G2. (b) Images from a high-throughput assay to identify G2 that decreases the actin-bundling function of fascin. (c) The dose–response curve for G2 from one high-throughput assay. (d) G2 had no effect on the actin-bundling activity of L-plastin (another actin-bundling protein). The dotted line was a linear fit of the data. (e) The effect of G2 on the actin-bundling activity of fascin assayed by the low-speed co-sedimentation assay. (f) Dose response of the inhibition of fascin function by G2 from the low-speed co-sedimentation assay. (g) Pre-incubation of fascin with G2 (25 μM) was not a pre-requirement for its inhibitory effect on fascin. Pre-incubation of fascin with G2 [(F+G2)+A], mixture of three components together (F+A+G2), or addition of G2 to the pre-formed fascin and actin bundles [(F+A)+G2], decreased the actin-fascin bundles. The control was with solvent used to dissolve G2. (h) Quantification of data ing. Data are representative of three similar experiments. Error bars, mean±s.e.m. of triplicates. Scale bars, 25 μm. Figure 2: Inhibition of the actin-bundling function of fascin by G2. ( a ) Chemical structure of G2. ( b ) Images from a high-throughput assay to identify G2 that decreases the actin-bundling function of fascin. ( c ) The dose–response curve for G2 from one high-throughput assay. ( d ) G2 had no effect on the actin-bundling activity of L-plastin (another actin-bundling protein). The dotted line was a linear fit of the data. ( e ) The effect of G2 on the actin-bundling activity of fascin assayed by the low-speed co-sedimentation assay. ( f ) Dose response of the inhibition of fascin function by G2 from the low-speed co-sedimentation assay. ( g ) Pre-incubation of fascin with G2 (25 μM) was not a pre-requirement for its inhibitory effect on fascin. Pre-incubation of fascin with G2 [(F+G2)+A], mixture of three components together (F+A+G2), or addition of G2 to the pre-formed fascin and actin bundles [(F+A)+G2], decreased the actin-fascin bundles. The control was with solvent used to dissolve G2. ( h ) Quantification of data in g . Data are representative of three similar experiments. Error bars, mean±s.e.m. of triplicates. Scale bars, 25 μm. Full size image To further confirm the inhibitory effect of G2 on the actin-bundling activity of fascin, we used a different and complementary approach of low-speed co-sedimentation assay, in which fascin would pellet together with the actin bundles ( Fig. 2e ). With increasing concentrations of G2, the fraction of actin and fascin proteins in the pellets was decreased, whereas the percentage of actin and fascin proteins in the supernatant was increased (IC 50 , ∼ 5 μM; Fig. 2e,f ). Furthermore, pre-incubation of fascin with G2 was not a pre-requirement. Preformation of actin bundles with fascin with subsequent addition of G2, or addition of G2 to the mixture of fascin and actin proteins also decreased the actin-fascin bundles, indicating that G2 could break preformed actin-fascin bundles ( Fig. 2g,h ). Together, these data confirm that G2 inhibits the actin-bundling function of fascin. Biochemical mechanism by which G2 inhibits fascin To understand the biochemical mechanism by which fascin inhibitors block the actin-bundling function of fascin, we investigated whether these inhibitors directly bind to fascin. During our screening of chemical libraries to identify the small-molecule inhibitors, we used a functional assay for fascin, namely, the actin-bundling activity of fascin. To confirm that they indeed directly bound to fascin, we used the isothermal titration calorimetry (ITC) technique and measured the direct interaction of fascin and the fascin inhibitor hits. ITC is a direct measurement of the heat generated or absorbed when molecules interact. It is used to determine the thermodynamic parameters of interactions of molecules (most often between small molecules and proteins) in solution. The experimental raw data consist of a series of spikes of heat flow (with every spike corresponding to one G2 injection). These spikes are then integrated with respect of time. The pattern of these heat effects as a function of the molar ratio [G2]/[fascin] could then be analysed to give the thermodynamic parameters of the interaction (see Methods). ITC assay revealed that G2 could directly interact with fascin ( Fig. 3a,b ). The K d was 5–20 μM and the stoichiometry was ∼ 1 ( Fig. 3b ). 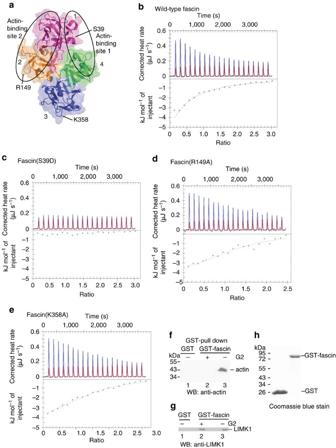Figure 3: Direct binding of G2 to fascin. (a) Diagram of the fascin structure showing the positions of fascin mutants fascin(S39D), fascin(R149A) and fascin(K358A). Fascin has four β-trefoil domains (labelled from 1 to 4, and in different colours). The two main actin-binding sites are marked. (b) Isothermal titration calorimetry assay shows the direct binding of G2 to wild-type fascin. (c) G2 does not interact with fascin(S39D). (d,e) G2 still interacts with Fascin(R149A) (d) and fascin(K358A) (e). (f) In GST-pull-down assays, G2 blocked the interaction of fascin and actin. Protein molecular mass markers are indicated on the left. (g) G2 had no effect on the interaction of fascin and LIMK1. Different amounts of whole-cell extracts from the same batch of cells treated with or without G2 were used infandg. (h) Coomassie Blue staining of purified GST and GST–fascin proteins used in GST-pull-down assays. Data are representative of three similar experiments. Figure 3: Direct binding of G2 to fascin. ( a ) Diagram of the fascin structure showing the positions of fascin mutants fascin(S39D), fascin(R149A) and fascin(K358A). Fascin has four β-trefoil domains (labelled from 1 to 4, and in different colours). The two main actin-binding sites are marked. ( b ) Isothermal titration calorimetry assay shows the direct binding of G2 to wild-type fascin. ( c ) G2 does not interact with fascin(S39D). ( d , e ) G2 still interacts with Fascin(R149A) ( d ) and fascin(K358A) ( e ). ( f ) In GST-pull-down assays, G2 blocked the interaction of fascin and actin. Protein molecular mass markers are indicated on the left. ( g ) G2 had no effect on the interaction of fascin and LIMK1. Different amounts of whole-cell extracts from the same batch of cells treated with or without G2 were used in f and g . ( h ) Coomassie Blue staining of purified GST and GST–fascin proteins used in GST-pull-down assays. Data are representative of three similar experiments. Full size image To determine the binding region of G2 on fascin, we took advantage of mutant fascin proteins that we previously generated. Others and we previously solved the X-ray crystal structure of fascin [35] , [45] , [46] . Based on the crystal structure, we generated 100 mutations of surface-exposed residues on fascin, and determined the actin-bundling and actin-binding activity of these 100 mutants [44] . The residues that were critical for actin-bundling activity were clustered in three regions and may represent different actin-binding sites on fascin ( Fig. 3a ). Therefore, we selected fascin mutants fascin(S39D), fascin(R149A) and fascin(K358A) from each of these three regions to study their interactions with G2 ( Fig. 3a ). The X-ray crystal structures of fascin mutants from these three regions showed that all these fascin mutants have the same structure (the inactive configuration), which is slightly different from that of the active configuration of wild-type fascin [44] . Thus, these mutations did not introduce major overall structural changes on fascin proteins. Although fascin(R149A) and fascin(K358A) still bound to G2 ( K d of ∼ 20 μM), fascin(S39D) did not ( K d > ∼ 200 μM; Fig. 3c–e ). Together, these data demonstrate that G2 directly interacts with fascin, and that G2 binds to the region around S39. These data also indicate that G2 binds to one of the actin-binding sites (including the residue S39) and thus likely interferes with the binding of actin filaments. Therefore, these data immediately reveal a potential mechanism of action for G2: this inhibitor occupies the actin-binding site 1, prevents the binding of actin filaments to this actin-binding site, and thus leads to the inhibition of the bundling activity of fascin. In addition to directly binding to actin filaments, fascin also directly interacts with other proteins including LIMK [47] , [48] , [49] . To investigate whether G2 could also interfere the interaction of fascin with these proteins, we performed the glutathione S -transferase (GST)-pull-down experiments with GST–fascin fusion protein and whole-cell lysates in the absence and presence of G2 ( Fig. 3f–h ). Although G2 blocked the interaction of fascin with actin ( Fig. 3f ), G2 did not affect the interaction of fascin with LIMK1 ( Fig. 3g ). The purity of purified GST and GST–fascin proteins used for the GST-pull-down assays was shown in Fig. 3h . These data further confirm the specific inhibitory effect of G2 on the actin-bundling function of fascin. G2 inhibition of fascin function in cells Next, we investigated the inhibitory effect of G2 on fascin activity in cells. As fascin is the main actin-bundling protein in filopodia, we examined whether G2 interfered with the formation of filopodia. To directly test this cell biological effect, we transfected fascin-green fluorescent protein (GFP) into MDA-MB-231 human metastatic breast tumour cells to visualize fascin-dependent filopodial formation. Filopodia containing GFP-fascin were quantified in terms of numbers of filopodia and the length of filopodia [44] . As we previously showed that, while GFP alone did not produce any GFP-containing filopodia, GFP-fascin induced the formation of GFP-fascin-containing filopodia [44] . Treatment with G2 decreased the number of filopodia per cell by about threefold ( Fig. 4a,b ). In addition, there were changes in cell shapes that G2 treatment led to rounded cells. Similar results were obtained with 4T1 mouse metastatic mammary tumour cells ( Fig. 4c,d ) and MCF-10A human mammary epithelial cells ( Fig. 4e,f ) when fascin-GFP was used to label the filopodia, as well as untransfected 4T1 cells when endogenous filopodia were stained with anti-fascin antibody ( Fig. 4g and Supplementary Fig. 1a ). Furthermore, we identified fascin(E391A) mutant that retained the actin-bundling activity but was insensitive to G2 inhibition ( Supplementary Fig. 1b ). After transfected into 4T1 cells, GFP-fascin(E391A) induced filopodial formation, which was resistant to G2 inhibition ( Supplementary Fig. 1c ). 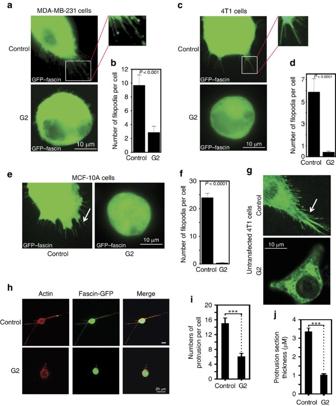Figure 4: G2 inhibits fascin activity in cells. (a) Inhibition of G2 on the filopodial formation. MDA-MB-231 cells were transfected with fascin-GFP and imaged by fluorescence microscopy. An enlarged image on the right shows the filopodia. (b) Quantification of data from experiments ina. The number of fascin-GFP-labelled filopodia per cell was counted;n=15. (c) 4T1 cells were transfected with fascin-GFP, treated with or without G2 and imaged by fluorescence microscopy. An enlarged image on the right shows the filopodia. (d) Quantification of data from experiments inc. The number of fascin-GFP-labelled filopodia per cell was counted;n=10. (e) MCF-10A cells were transfected with fascin-GFP, treated with or without G2 and imaged by fluorescence microscopy. (f) Quantification of data from experiments ine. The number of fascin-GFP-labelled filopodia per cell was counted;n=14. (g) Untransfected 4T1 cells, treated with or without G2, were stained with anti-fascin antibody and imaged by fluorescence microscopy. (h) G2 treatment decreased the number of membrane protrusions of MDA-MB-231 cells in collagen gel. 3D reconstruction from confocal image sections from cell expressing fascin-GFP with or without the G2 inhibitor. (i,j) Fascin inhibition with G2 affects the average number of protrusion per cells (i) and protrusion thickness (j). Bars denote s.e.m. Statistical analysis was done with Student’st-test. ***P<0.001. Figure 4: G2 inhibits fascin activity in cells. ( a ) Inhibition of G2 on the filopodial formation. MDA-MB-231 cells were transfected with fascin-GFP and imaged by fluorescence microscopy. An enlarged image on the right shows the filopodia. ( b ) Quantification of data from experiments in a . The number of fascin-GFP-labelled filopodia per cell was counted; n =15. ( c ) 4T1 cells were transfected with fascin-GFP, treated with or without G2 and imaged by fluorescence microscopy. An enlarged image on the right shows the filopodia. ( d ) Quantification of data from experiments in c . The number of fascin-GFP-labelled filopodia per cell was counted; n =10. ( e ) MCF-10A cells were transfected with fascin-GFP, treated with or without G2 and imaged by fluorescence microscopy. ( f ) Quantification of data from experiments in e . The number of fascin-GFP-labelled filopodia per cell was counted; n =14. ( g ) Untransfected 4T1 cells, treated with or without G2, were stained with anti-fascin antibody and imaged by fluorescence microscopy. ( h ) G2 treatment decreased the number of membrane protrusions of MDA-MB-231 cells in collagen gel. 3D reconstruction from confocal image sections from cell expressing fascin-GFP with or without the G2 inhibitor. ( i , j ) Fascin inhibition with G2 affects the average number of protrusion per cells ( i ) and protrusion thickness ( j ). Bars denote s.e.m. Statistical analysis was done with Student’s t -test. *** P <0.001. Full size image In vivo , filopodia function as cell’s sensory organs and communicate with the extracellular environment. To study the effect of G2 on filopodial formation in a 3D environment, we performed live-cell imaging study of MDA-MB-231 cells transfected with fascin-GFP in a 3D environment with collagen gel ( Fig. 4h–j ). We should note that, in tumour cells, these finger-like membrane protrusions are sometimes called invadopodia [50] , [51] . For simplicity, here we referred them as membrane protrusions. Although untreated cells had long and multiple membrane protrusions ( Fig. 4h ), G2-treated cells were with much shorter and fewer membrane protrusions ( Fig. 4h,i ). In addition, the thickness of the protrusions was decreased by G2 treatment ( Fig. 4j ). This effect is similar to what we observed in the HTS assay ( Fig. 2b ). Together, these data demonstrate that G2 inhibits fascin function in cells and impairs the filopodial formation. Fascin inhibitor blocks tumour cell migration and invasion To further investigate the cellular biological effect of G2, we studied the migration of tumour cells in the absence or presence of G2 using the quantitative Boyden chamber assay. G2 inhibited the migration of both MDA-MB-231 human metastatic breast tumour cells and 4T1 mouse metastatic mammary carcinoma cells ( Fig. 5a–d ). G2 had no effect on the growth of MDA-MB-231 and 4T1 tumour cells, as shown by the soft agar colony formation assay ( Fig. 5e,f ). The number of colonies in G2-treated and untreated groups was similar ( Fig. 5f ). We noticed that colonies formed by untreated cells were with rough surface and that those formed by G2-treated cells were with smooth surface, which might contribute to the slightly smaller sizes of these colonies ( Fig. 5e ). The size differences were consistent with that G2 treatment blocked filopodial formation and caused cell rounding ( Fig. 4 ). G2-treated cells might also have a survival disadvantage in soft agar. Furthermore, G2 did not induce apoptosis of either MDA-MB-231 cells or 4T1 cells ( Fig. 5g ). Together, these data demonstrate that G2 could inhibit breast tumour cell migration specifically. 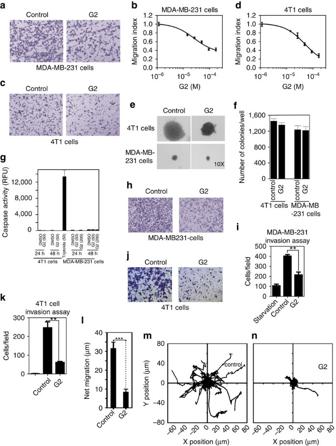Figure 5: Inhibitory effect of G2 on breast tumour cell migration and invasion. (a) Inhibition of the migration of MDA-MB-231 cells by G2 in response to serum stimulation as shown by Boyden-chamber assay. (b) Dose–response curve for the inhibition of the migration of MDA-MB-231 cells by G2. Error bars, mean±s.e.m. of triplicates. (c) Inhibition of the migration of 4T1 cells by G2 in response to serum stimulation. (d) Dose–response curve for the inhibition of the migration of 4T1 cells by G2. (e,f) Soft-agar colony formation assay showed that no effects on the growth of MDA-MB-231 cells or 4T1 cells by G2. Data are mean±s.e. of three experiments. (g) G2 did not induce apoptosis of MDA-MB-231 cells or 4T1 cells. Cells were treated with the control DMSO or G2 (50 or 200 μM). Theyaxis values correspond to the relative fluorescent unit (RFU) as a measure of caspase activity using a fluorescence-based caspase-3 substrate. Error bars are s.e.m. of three independent assays. Triptolide (50 μM) is known to induce apoptosis and used as a positive control. (h) Inhibition of MDA-MB-231 cell invasion by G2 in response to serum stimulation as shown by the matrigel invasion assay. (i) Quantification of data inh. (j) Inhibition of 4T1 cell invasion by G2 in response to serum stimulation. (k) Quantification of data inj. (l–n) MDA-MB-231 cells average net migration in 1.5 mg ml−1collagen gels measured over 20 h with or without G2 along with the corresponding tracks. Data are representative of three similar experiments. Error bars, mean±s.e.m. Statistical analyses were done with Student’st-test. **P<0.05. ***P<0.001. Scale bars, 100 μm. Figure 5: Inhibitory effect of G2 on breast tumour cell migration and invasion. ( a ) Inhibition of the migration of MDA-MB-231 cells by G2 in response to serum stimulation as shown by Boyden-chamber assay. ( b ) Dose–response curve for the inhibition of the migration of MDA-MB-231 cells by G2. Error bars, mean±s.e.m. of triplicates. ( c ) Inhibition of the migration of 4T1 cells by G2 in response to serum stimulation. ( d ) Dose–response curve for the inhibition of the migration of 4T1 cells by G2. ( e , f ) Soft-agar colony formation assay showed that no effects on the growth of MDA-MB-231 cells or 4T1 cells by G2. Data are mean±s.e. of three experiments. ( g ) G2 did not induce apoptosis of MDA-MB-231 cells or 4T1 cells. Cells were treated with the control DMSO or G2 (50 or 200 μM). The y axis values correspond to the relative fluorescent unit (RFU) as a measure of caspase activity using a fluorescence-based caspase-3 substrate. Error bars are s.e.m. of three independent assays. Triptolide (50 μM) is known to induce apoptosis and used as a positive control. ( h ) Inhibition of MDA-MB-231 cell invasion by G2 in response to serum stimulation as shown by the matrigel invasion assay. ( i ) Quantification of data in h . ( j ) Inhibition of 4T1 cell invasion by G2 in response to serum stimulation. ( k ) Quantification of data in j . ( l – n ) MDA-MB-231 cells average net migration in 1.5 mg ml −1 collagen gels measured over 20 h with or without G2 along with the corresponding tracks. Data are representative of three similar experiments. Error bars, mean±s.e.m. Statistical analyses were done with Student’s t -test. ** P <0.05. *** P <0.001. Scale bars, 100 μm. Full size image We next investigated the effect of G2 on tumour cell invasion with two different assays. First, we used a Matrigel invasion assay, which requires the tumour cells to invade through a 3D matrix to reach the bottom of the chamber ( Fig. 5h–k ). Serum induced the invasion of MDA-MB-231 human breast tumour cells ( Fig. 5h,i ). Addition of G2 inhibited the serum-induced tumour cell invasion ( Fig. 5h,i ). Furthermore, we observed similar inhibitory effect of G2 on the invasion of 4T1 mouse breast tumour cells ( Fig. 5j,k ). Then, we used live-cell imaging to track the invasion/movement of MDA-MB-231 cells in a 3D environment with collagen gel ( Fig. 5l–n ). In the absence of G2, MDA-MB-231 cells had a net migration of ∼ 32 μm over a 24-h period ( Fig. 5l ). On the other hand, G2-treated MDA-MB-231 cells moved a net distance of ∼ 8 μm ( Fig. 5l ). Moreover, untreated MDA-MB-231 cells explored much broader area than G2-treated cells ( Fig. 5m,n ). Therefore, G2 inhibits tumour cell invasion in 3D matrices. Inhibition of tumour metastatic colonization by G2 We further investigated the effect of fascin inhibitors on tumour metastatic colonization in animal models. The pharmacokinetics of G2 were analysed in mice. Serum concentrations of G2 were determined using liquid chromatography coupled to tandem mass spectrometry. G2 showed properties that define a good drug candidate ( Supplementary Fig. 2a and b ). We used two mouse models to test the effect of G2 on tumour metastasis. In the first orthotropic spontaneous tumour metastasis mouse model, 4T1 mouse breast tumour cells were injected into the orthotropic site (the mammary gland) and then the metastasis to the lung was monitored [35] , [52] , [53] ( Fig. 6a ). The 4T1 mouse tumour closely mimics human breast cancer in its anatomical site, immunogenicity, growth characteristics and metastatic properties [54] . From the mammary gland, the 4T1 tumour spontaneously metastasizes to a variety of target organs including lung, bone, brain and liver. Previously, we demonstrated that fascin-shRNA-expressing 4T1 (and MDA-MB-231) tumour cells had lower metastasis than control-shRNA-expressing cells [35] . Seven days after implantation of 4T1 tumour cells, we injected the mice with control solvent or G2 (daily at 100 mg kg −1 ). After 18 days, the mice were killed and examined for metastasis in the lungs [35] , [52] , [53] . Whereas mice injected with control solvent exhibited large numbers of metastasized 4T1 cells in the lungs, the number of metastasized 4T1 cells in the lungs of mice treated with G2 was reduced by ∼ 95% ( Fig. 6a ). In similar experiments, we observed that G2 treatment had no significant effect on the growth of primary tumours ( Supplementary Fig. 2 c and d ), and that G2 reduced the number of tumour nodules in the lung ( Supplementary Fig. 2e ). Furthermore, metastasis of fascin shRNA-treated 4T1 cells with re-expression of human fascin(E391A) mutant was insensitive to G2 ( Supplementary Fig. 2e ). These results demonstrate that G2 is a potent inhibitor of 4T1 tumour cell metastasis from the mammary gland to the lungs, and the actin-bundling activity as well as filopodia are critical for tumour metastasis in mouse models. 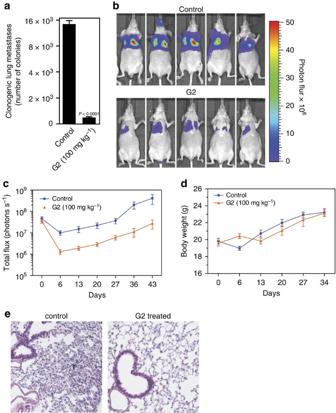Figure 6: Inhibitory effect of G2 on breast tumour lung colonization. (a) Inhibition of 4T1 mouse mammary tumour cell metastasis to the lung by G2 in a spontaneous metastasis model (n=5). (b,c) Inhibition of lung colonization by G2 in a mouse model. Control group (n=8) was treated with saline. G2 (100 mg kg−1) was used for the treatment group (n=9). Representative IVIS images are shown inb. (d) G2 had no effect on the body weights of treated mice. Error bars, mean±s.e.m. (e) Histological analyses (haematoxylin and eosin staining) show lung tissue sections from mice injected with MDA-MB-231 cells treated with control solvent or treated with G2. ‘T’ indicates tumour metastases. Data are representative of three similar experiments. Scale bars, 100 μm. Figure 6: Inhibitory effect of G2 on breast tumour lung colonization. ( a ) Inhibition of 4T1 mouse mammary tumour cell metastasis to the lung by G2 in a spontaneous metastasis model ( n =5). ( b , c ) Inhibition of lung colonization by G2 in a mouse model. Control group ( n =8) was treated with saline. G2 (100 mg kg −1 ) was used for the treatment group ( n =9). Representative IVIS images are shown in b . ( d ) G2 had no effect on the body weights of treated mice. Error bars, mean±s.e.m. ( e ) Histological analyses (haematoxylin and eosin staining) show lung tissue sections from mice injected with MDA-MB-231 cells treated with control solvent or treated with G2. ‘T’ indicates tumour metastases. Data are representative of three similar experiments. Scale bars, 100 μm. Full size image In the second experimental metastasis mouse model, MDA-MB-231 human breast tumour cells were retrovirally infected with a triple-fusion protein reporter construct encoding herpes simplex virus thymidine kinase 1, GFP and firefly luciferase [53] , [55] . These cells were injected into the tail vein of immuno-deficient mice (NOD-SCID mice). The extravasation and lung colonization of tumour cells were monitored by non-invasive bioluminescence imaging [35] , [52] , [53] ( Fig. 6b,c ). In the control group, the solvent was injected. In the treatment group, G2 was intraperitoneally injected. Progressively increasing signals after 6 days in mice with control solvent-treated mice indicated that cells had succeeded in colonization and proliferating [35] ( Fig. 6c ). When given daily to mice with injected MDA-MB-231 tumour cells, G2 treatment (100 mg per kg of weight (mg kg −1 )) reduced the tumour colonization in lungs by ∼ 95% ( Fig. 6b,c ). Treatment was tolerated well with no signs of toxicity during 6 weeks of daily treatment ( Fig. 6d ). Furthermore, lung tissues from the control group showed many MDA-MB-231 tumour cells, whereas lung tissues from G2-treated group had much lower number of tumour cells ( Fig. 6e ). Together, these data demonstrate that G2 can markedly decrease the lung colonization of breast tumour cells in animal models, and the importance of filopodia in metastatic colonization. Toxicity study of G2 in mice To assess toxicity of G2 in mice, athymic mice were dosed with either control vehicle (dimethylsulphoxide (DMSO)) or 100 mg kg −1 G2 compound i.p. daily, 5 days per week, for 2 weeks, at which point all animals were killed and processed for histopathology. All mice survived to the end of the study, looked healthy, behaved normally and maintained a normal, healthy, body weight throughout the study ( Fig. 7a ). At time of killing (day 15) the mice, blood was collected for clinical chemistry analysis, and complete necropsy was performed on all mice. Clinical chemistry parameters from both groups were within normal range ( Fig. 7b ), with the exception of elevated liver enzymes (alanine transaminase and aspartate aminotransferase) and decreased albumin levels, with no statistically significant difference between the G2 treated and the corresponding controls. This was most likely due to inflammatory response to repeated dosing with the vehicle (DMSO) and not related to G2 specifically. 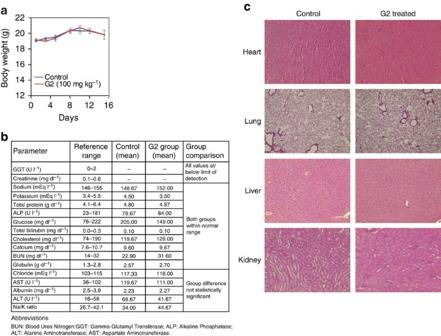Figure 7: Toxicity study of G2 in mice. (a) G2 had no effect on the body weights of treated mice. Error bars, mean±s.e.m. (b) Clinical chemistry of blood samples from all mice from the control and G2-treated groups. (c) Histopathological analyses (hematoxylin and eosin staining) of some major organs show no specific toxic effects of G2. Scale bar, 100 μm. Figure 7: Toxicity study of G2 in mice. ( a ) G2 had no effect on the body weights of treated mice. Error bars, mean±s.e.m. ( b ) Clinical chemistry of blood samples from all mice from the control and G2-treated groups. ( c ) Histopathological analyses (hematoxylin and eosin staining) of some major organs show no specific toxic effects of G2. Scale bar, 100 μm. Full size image Tissues from all mice were fixed, processed, embedded in paraffin, sectioned and stained with haematoxylin and eosin (H&E). Major organs, including the heart, lung, kidney, spleen, liver, pancreas, lymph nodes and intestines, were examined microscopically and no lesions were observed, with the exception of the liver ( Fig. 7c ), where multifocal mixed leukocytic infiltrates, indicative of an inflammatory response or cellular repair, were present in both G2-treated and control groups. Because all lesions observed in the livers of G2-treated mice were also found in the control group with similar incidence and severity, the hepatocellular injury was likely due to repeated dosing with the vehicle (DMSO) and not related to G2 specifically. Hence, 100 mg kg −1 daily G2 dosing in mice over a 2-week period did not result in any toxicity that was specifically attributed to G2. Elevated fascin expression is associated with increased risk of metastasis and mortality from patient studies, and increased numbers of filopodia are correlated to increased invasiveness, aggressivity and decreased survival rate [17] , [18] , [30] . To develop therapeutics for metastatic cancer treatment, we developed an HTS method, screened chemical libraries and identified small-molecule compounds that specifically inhibit the actin-bundling function of fascin. One of the small-molecule inhibitor G2 was further shown to inhibit the actin-bundling function of fascin, and blocks tumour cell migration, invasion and metastasis. We included a negative selection with another actin-bundling protein L-plastin to purposely look for inhibitors that specifically disrupt the fascin–actin filament interaction, and eliminated some small-molecule inhibitors for fascin which also inhibited the actin-bundling by L-plastin. Although it might be useful, in some cases, for a broad actin-bundling inhibitor, these inhibitors might be toxic to animals and human given that actin-bundling occurs in many cellular processes in addition to filopodia. The fascin-specific inhibitor is expected to be less toxic as fascin protein is normally not expressed in adult epithelial cells and most tissues/cells, and it is overexpressed in metastatic carcinomas. Furthermore, fascin knockout mice appear normal [33] . This is also consistent with our observation that mice injected with G2 for more than 2 months appeared normal with no evidence of weight loss, lethargy or ruffled fur. Toxicity study of G2 (at 100 mg kg −1 ) did not show any specific toxic effect in mice. Our intention of identifying fascin-specific inhibitor is further supported by the ITC data showing the direct interaction of G2 with fascin. Mechanistically, G2 binds directly to one of the actin-binding sites on fascin. Previously, we solved the X-ray crystal structures of wild-type fascin and four fascin mutants that are defective in actin-bundling activity [35] , [44] . The crystal structures of all these four fascin mutants have similar structures and thus define the inactive conformation [44] . When compared with the structure of the active wild-type fascin, the inactive fascin conformation has an overall similar structural folds with some minor configurational changes [44] . These data provide structural basis for the defects in actin-bundling by these fascin mutations, for the minor conformational changes for fascin from inactive to active states in the process of bundling actin filaments, and for structure-based design of inhibitors that stabilize the inactive conformation of fascin. Furthermore, these structural data provide a mechanistic explanation for the cooperativity among the actin-binding sites [44] . It has been shown that the actin-binding activity of fascin is cooperative [56] . Our data reveal that fascin mutants in all actin-binding sites display the same inactive configuration. This indicates that any impairment in one actin-binding site leads to a concerted conformational change, thus disable the other actin-binding sites. The actin-binding sites are conformationally interconnected. Hence, it is likely that binding of one F-actin filament at one actin-binding site stabilizes fascin at the active configuration and enhances the binding of actin filaments at the other actin-binding sites. Therefore, we speculate that G2 binding at one actin-binding site stabilizing fascin at its inactive conformation, leading to the inhibition of its actin-bundling activity. Fascin is a biomarker of some metastatic carcinomas. We and others have shown that breast tumour samples from patients showed elevated fascin expressions comparing to normal samples [35] . We found that the levels of fascin transcripts were significantly higher in triple-negative breast tumours [35] . Overexpression of fascin contributes to a more aggressive clinical course of cancer [32] . Kaplan–Meier analyses showed that higher fascin expression was associated with lower overall survival and lower metastasis-free survival [35] . These data highlight the correlation between higher fascin expression and metastasis and death in human breast cancer patients. In addition to breast cancers, elevated levels of fascin have been found in other metastatic tumours and are correlated with clinically aggressive phenotypes, poor prognosis and shorter survival [32] , [37] , [38] , [41] , [42] , [43] . Although there are several different actin-cross-linker proteins, fascin is specifically overexpressed in many types of metastatic tumour cells [37] , [38] , [39] , [40] . Fascin is also one of the gene signatures that correlate with breast cancer metastasis to the lung [57] . A recent systematic review and meta-analysis of 26 immunohistochemical studies (total ∼ 9,000 patients) of the five prevalent human carcinomas (breast, colorectal, gastric, lung and oesophageal carcinomas) revealed that, in breast, colorectal and oesophageal carcinomas, high levels of fascin are associated with increased risk of mortality and disease progression [30] . Pooled analysis of all carcinomas indicate that high levels of fascin are associated with increased risk of mortality, lymph node metastasis and distant metastasis, and may provide a novel biomarker for early diagnosis of aggressive and metastatic tumours [30] . Furthermore, another systematic review and meta-analysis of resected cholangiocarcinoma from 73 immunohistochemical studies (total 4,126 patients) uncovered several biomarkers prognostic of overall survival consisting of fascin, EGFR, MUC1, MUC4 and p27 (ref. 58 ). These predictive biomarkers may allow for personalized cancer treatment, and such biomarkers could serve as targets for anticancer therapy. Moreover, a recent study of serum levels of fascin proteins from non-small-cell lung cancer patients and healthy volunteers shows that the serum fascin protein level is markedly increased in the cancer patients, particularly in advanced cases (stage III or IV), compared with that in the healthy controls [59] . The serum fascin level reflects the aggressive progress of both lymphatic and distant metastasis, and is an independent prognostic factor [59] . Most current treatments for metastatic cancers are aimed to kill or stop the growth of primary cancer cells and metastatic cancer cells. Even though tumour cell migration and invasion are critical steps in the process of tumour metastasis, specific inhibitors of tumour cell migration have not been used in the current treatment for metastatic cancers. Therefore, it is desirable to develop small-molecule inhibitors targeting tumour cell migration as novel methods for treating breast cancer. Furthermore, microtubule protein tubulin has been successfully used as a drug target for decades. Yet no actin cytoskeletal proteins have been clinically used as therapeutic targets for cancer treatment. Our studies of fascin as a good therapeutic target for anti-metastatic agents raise the potential of using actin cytoskeletal proteins such as fascin as novel targets for cancer treatment, in a similar manner to the microtubule protein tubulin. Moreover, future combinatory uses of anti-growth and anti-metastatic agents should significantly improve the survival of cancer patients. Mouse colony NOD-SCID immunodeficient mice (female 6- to 8–week-old) were purchased from the Jackson Laboratory. Studies using mice were performed in compliance with the Institutional Animal Care and Use Committee of Weill Medical College of Cornell University. All mice were housed in the facility of the Research Animal Resource Center of Weill Medical College of Cornell University. Cell culture Mouse 4T1 mammary tumour cells and human MDA-MB-231 breast tumour cells were obtained from American Type Culture Collection. 4T1 cells were cultured in RPMI 1640 medium supplemented with 10% fetal bovine serum (FBS). MDA-MB-231 cells were cultured in DMEM supplemented with 10% FBS. Human fascin-1 expression and purification Recombinant human fascin 1 was expressed as a GST fusion protein in BL21 Escherichia coli . One-litre of 2YT medium with ampicillin was inoculated overnight with 3 ml of BL21/DE3 culture transformed with pGEX4T-fascin 1 plasmid and grown at 37 °C until attenuance at 600 nm (OD 600 ) reached about 0.5. The culture was then transferred to 17 °C and induced by the addition of 0.1 mM isopropyl β- D -thiogalactoside for 16 h. Bacteria were harvested by centrifugation at 5,000 r.p.m. for 10 min. The pellets were suspended in 30 ml of Tris-HCl (20 mM Tris-HCl, pH 8.0, 150 mM NaCl) supplemented with 0.2 mM phenylmethylsulphonyl fluoride, 1 mM dithiothreitol (DTT), 1 % Triton X-100 and 1 mM EDTA. After sonication, the suspension was centrifuged at 15,000 r.p.m. for 30 min to remove the cell debris. The supernatant was then incubated for 2 h with 4 ml of glutathione beads (Sigma) at 4 °C. After extensive washing with Tris-HCl (20 mM Tris-HCl pH 8.0, 150 mM NaCl), the beads were resuspended in 10 ml of thrombin cleavage buffer (20 mM Tris-HCl, pH 8.0, 150 mM NaCl, 2 mM CaCl 2 , 1 mM DTT). Fascin was released from the beads by incubation overnight with 40–100 U of thrombin at 4 °C. After centrifugation, 0.2 mM phenylmethylsulphonyl fluoride was added to the supernatant to inactivate the remnant thrombin activity. The fascin protein was further concentrated with Centricon to about 50 mg ml −1 . Chemical library screens and analysis The low-speed co-sedimentation assay was generally used to probe the actin-bundling activity of fascin in vitro . However, such assay is not practical to scale up in a high-throughput setting. We tried an AlphaScreen assay (a luminescence based assay to detect protein-protein interaction) and an actin polymerization assay (based on the enhanced fluorescence of pyrene-conjugated actin that occurs during polymerization). These two approaches did not show promise. We then developed an imaging-based assay where we could observe the fascin-mediated actin bundles. Chemical library screening was conducted at the High-Throughput Screening Resource Center at Rockefeller University. A total of ∼ 150,000 compounds were screened. These chemical compounds were from the LOPAC 1280 collection, the Prestwick chemical library, the Pharmakon collection, the MicroSource Spectrum collection, the Life Chemicals library, the Greenpharma natural compound library, the Enamine library, the ChemBridge library, the Chem-X-Infinity library and the BioFocus DPI library. Fifteen microlitres of 0.5 μM purified fascin protein in buffer (100 mM KCl, 20 mM Tris-HCl, pH 7.5, 2 mM MgCl 2 ) was added into each well of a clear 384-well flat-bottom plate (Corning) using Thermo Multidrop Combi (Fisher). A volume of 180 nl of compound solutions (5 mM stock) from various chemical libraries were pin transferred from stock 384-well plates into the 384-well assay plates and was incubated for 30 min. Then 15 μl of 0.5 μM polymerized actin (in 100 mM KCl, 20 mM Tris-HCl, pH 7.5, 2 mM MgCl 2 , 1 mM DTT, 1 mM ATP; Cytoskeleton Inc.) was added, resulting in ∼ 30 μM final concentration for chemical compounds. After another 30 min, 10 μl of Alexa Fluro-488 Phalloidin (25 times dilution from stocks in 100% methanol, Invitrogen) was added to stain F-actin and was incubated in the dark for 1 h. Twenty-five microlitres of the mixed solution were then transferred to one well in a black 384-well plate coated with poly- D -lysine, and stained actin bundles or F-actin would stick onto the poly- D -lysine plates. After thoroughly washed with PBS for three times, the plate was imaged at the Weill Cornell Cell Screening Facility using an ImageXpress Micro High Content Screening System (Molecular devices). The negative control wells were employed for quality control: multiple DMSO-only control wells (16 wells per plate) were present on each assay plate. Two criteria were used to filter the desired compounds: z-score was less than −3 and the images look like the image of actin alone. In the confirmative screens, ∼ 700 compounds were tested in duplicates. In all, 145 compounds with confirmed responses were picked and preceded to the IC 50 studies. The Z’ factor was 0.5012 for the average fibre length, and 0.5908 for the average fibre breadth, indicating this was a robust assay that was suitable for HTS. G2 source and chemical characterization Compound G2 was initially purchased from BioFocus. The compound purity was 96%. Molecular weight of 385.344. G2 was later resynthesized by ValueTek Inc. 1 H NMR (400 MHz, CHLOROFORM-d) δ =8.73 (s, 1H), 8.09–8.30 (m, 1H), 7.50–7.59 (m, 3H), 7.35–7.43 (m, 1H), 7.24–7.33 (m, 4H), 7.17 (ddd, J =0.88, 6.99, 8.20 Hz, 1H), 6.58 (dd, J =1.76, 3.52 Hz, 1H), 5.54 (s, 2H). MS (ESI) m/z : 414 (M+H)+. HRMS (ESI) calcd for C20H15F3N3O2 (M+H)+ m / z =386.1018, found 386.1016. High-content image acquisition and analysis An ImageXpress MICRO imaging system from Molecular Devices equipped with a 300-W Xenon-arc lamp from Perkin-Elmer, a Nikon × 40 Plan Fluor 0.6 numerical aperture (NA) objective, and a Photometrics CoolSnapHQ camera (1,392 × 1,040 pixels) from Roper Scientific was used to acquire images. Alexa Fluor 488 images were acquired using 482/35 nm excitation and 536/40 nm emission filters with a 513 dichroic long-pass filter obtained from Semrock. Plates were transported from plate hotels using a CRS CataLyst Express robot from Thermo Scientific. Images were acquired at four sites per well, with 1,200 ms exposure time per image using 2 × 2 binning. Each site was individually focused using a high-speed laser autofocus comprised of a 690-nm diode laser and a dedicated 8-bit CMOS camera. Acquisition time was 90 min per plate. 696 × 520 pixel images were acquired at 12 intensity bits per pixel. Each pixel is 0.3225 × 0.3225 μm 2 in the object. Images were analysed using MetaXpress image-analysis software from Molecular Devices. To correct for shading, a shading image was created by averaging all of the images from a plate and smoothing the averaged image using a median filter. Then each pixel in an image was multiplied by the average intensity of the shading image and the resulting pixel intensities were divided by the shading image on a pixel-by-pixel basis. Background was subtracted from each shading-corrected image by multiplying the pixels intensities by two then determining the fifth percentile intensity value of the resulting image and subtracting this value from each pixel in the image. Finally, an Unsharp Mask was applied to minimize out of focus blur in the image. The processed image was thresholded in order to segment the objects of interest from the background. The Integrated Intensity and the Percent Threshold Area of the thresholded image were measured using the Show Region Statistics function of MetaXpress. Object Count, Fibre Length and Fibre Breadth were measured using the Integrated Morphometry Analysis function of MetaXpress. The sum of each measurement for the four sites per well was divided by the number of sites to get the average measurement per well. All image processing and measurement steps were done automatically on each image using a custom journal, which also recorded the measurements to an Excel spreadsheet. The Z-factor was calculated based on the following formula: The σ p and σ n are the standard deviations of the positive (p) and negative (n) controls, and μ p and μ n are the means of the positive and negative controls. HTS data were managed using Collaborative Drug Discovery software and R program. F-actin bundling assay Actin-bundling activity was measured by low-speed centrifugation assay and fluorescence microscopy. In low-speed centrifugation assay, monomeric rabbit G-actin was induced to polymerize at room temperature in F-actin buffer (20 mM Tris-HCl at pH 8, 1 mM ATP, 1 mM DTT, 2 mM MgCl 2 and 100 mM KCl). Recombinant fascin proteins (wide-type or mutant) were subsequently incubated with F-actin for 30 min at room temperature and centrifuged for 15 min at 10,000 g in an Eppendorf 5415D table-top centrifuge. Both supernatants and pellets were dissolved in an equivalent volume of SDS sample buffer, and the amount of actin was determined by SDS-PAGE. We measured the intensities of fascin proteins in Coomassie-stained gels and then calculated the relative actin-bundling activity, P , by the following formula: P=100 × M p /M pc , where P is the relative actin-bundling activity, M p is the percentage of actin present in pellet when mixed with different concentrations of fascin protein, calculated by (intensity in pellet)/(intensity in pellet+intensity in supernatant), and M pc is the percentage of actin that is present in pellet when mixed with 0.25 μM fascin, which is used at a saturated concentration determined in our control experiment. In fluorescence microscopy, monomeric G-actin was polymerized as described earlier. F-actin was mixed with recombinant fascin protein in F-buffer (20 mM Tris-HCl at pH 8, 1 mM ATP, 1 mM DTT, 2 mM MgCl 2 and 100 mM KCl) and incubated at room temperature for 60 min. Actin was then labelled by adding 2% Alexa 488–phalloidin to the mixture. The samples were applied to a coverslip that was freshly coated with 1 mg ml −1 poly- D -lysine. After 60 min incubation, the coverslip was mounted on a slide and the image was taken on fluorescence microscopy. Three randomly selected fields (× 63 objectives) were photographed, and the bundles were counted. The Bundles/Field was expressed as the average number of bundles±s.d. Isothermal titration calorimetry Calorimetric measurements were carried out using a Low Volume Nano ITC instrument from the TA Instruments. In each experiment, the ligand was titrated to the protein solution present in the 500 μl sample cell. The reference cell contained 0.1 mM sodium azide dissolved in double-distilled water. All measurements were carried out at 25 °C. The protein was dissolved in 20 mM Tris-HCl buffer (pH 7.5), 100 mM NaCl to a concentration of 50 μM. Protein concentrations were determined by ultraviolet spectroscopy (280 nm) using the specific absorption calculated by the ProtParam tool. The ligand solution contained 1.2 mM of the corresponding inhibitor dissolved in the same buffer as the protein. Solutions were degassed at 25 °C under vacuum for 10 min. Upon experimental setup, the protein solution present in the sample cell was stirred at 320 r.p.m. After a stable baseline had been achieved, the titration was initiated. The injection sequence composed 20 injections of 2.4 μl in time intervals of 180 s until complete saturation was obtained. Heat changes caused by each inhibitor injection were obtained from the integral of the calorimetric signal. Data were analysed using the NanoAnalyze software (TA Instruments) for fitting points to the independent binding model. Experimental heats of the protein-inhibitor titration were corrected for heats of dilution by subtracting the average heat of the last three measurements after saturation of the protein-binding sites has occurred. All measurements were carried out at least in triplicate. Given energy values, binding constants and standard deviations were derived from data fitting and subsequent averaging of the corresponding measurements. Standard Gibbs free energy values were calculated using the equation Δ G 0 =- RT ln K b (where R =8.3144 J mol −1 K −1 , K b binding constant). GST-pull-down assay GST or GST–fascin proteins were expressed in BL21 cells and purified on glutathione-agarose beads. Whole-cell extracts of 4T1 cells (treated with or without 100 μM G2) were incubated with GST or GST–fascin proteins (5 μg) for 2 h at 4 °C. After washed three times with PBS+0.1% Triton X-100 to remove unbound proteins, bound proteins were resolved on SDS–PAGE, electroblotted onto nitrocellulose membrane and identified with anti-actin (Santa Cruz Biotechnology, sc-1616, 1:500 dilution) or anti-LIMK1 (Santa Cruz Biotechnology, sc-5576, 1:200 dilution) antibody. Signal was detected by chemiluminescence. Images in Fig. 3f,g were cropped for presentation. Full-size images are presented in Supplementary Fig. 3 . Fluorescence microscopy GFP-fascin-transfected cells were seeded onto laminin-coated glass coverslips in starvation condition (no serum) for 2 h with or without G2 (125 μM). Cells were fixed with 3.7% formaldehyde in PBS for 10 min at room temperature, permeabilized with 0.1% Triton X-100 for 5 min, and then washed three times with PBS. For untransfected 4T1 cells, anti-fascin monoclonal antibody (Santa Cruz Biotechnology) was used for immunofluorescent staining. The coverslips were then mounted onto slides and imaged using Zeiss LSM510 confocal microscopy. 3D cell migration Type I collagen was extracted from rat tail tendons (Pel-Freez Biologicals) via acid-solubilization, purified via centrifugation and lyophilization, and reconstituted in 0.1% acetic acid at 10 mg ml −1 . 100, 200 or 500 μl of the 10 mg ml −1 stock collagen solution was diluted up to 850 μl by gently mixing with 0.1% acetic acid on ice and neutralized to pH 7.0 with 100 μl of 1 M HEPES. 50 μl of MEM containing 50,000 MDA-MB-231 cells was then gently mixed with the collagen yielding a final collagen concentration of 1.5 mg ml −1 . A volume of 200 μl per wells of the gel solution were then poured into a glass-bottom 24-well plate (MatTek). Gels were the incubated at 37 °C for 45 min for collagen polymerization after which they were overlaid with 1.5 ml with or without G2 (125 μM) of pre-warmed culture media. Individual cell migration was observed with a wide-field digital imaging system (Zeiss Axio Observer Z1, Hamamatsu ORCA-ER camera and Axiovision software v. 4.8.1.0) equipped with an environmental chamber. Phase-contrast images were captured at 30 min intervals over a 24-h period, using a × 20/NA=0.5 ph2 dry objective. The cell locomotion was tracked using ImageJ software (v. 1.46, National Institutes of Health). Care was taken to ensure that these cells were at least 150 μm away from the bottom of the dish. Quantification of cell behaviour was obtained from at least three independent experiments and the different migration parameters are for at least 60 cells. The migration parameters were computed only for the XY imaging plane and cells moving too far out of focus were not analysed. Confocal cell imaging For actin imaging, the collagen gels were washed once with PBS, fixed for 10 min at room temperature (RT) with 3.7% formaldehyde in PBS, followed by methanol/acetone (3:7) for 5 min at −20 °C. Actin was stained with phalloidin-Alexa Fluor TexasRed (1/100 in PBS) at RT for 2 h on the rocker. Nuclei were stained with 4,6-diamidino-2-phenylindole (0.1 mg ml −1 in PBS) for 10 min at RT. Images were captured on a Zeiss LSM 700 microscope using the 450, 488 and 543 nm excitation laser lines and a × 40/1.1 NA objective water immersion objective and operated by Zen software (v. 2010, Carl Zeiss MicroImaging GmbH). 3D image reconstruction and quantification of cell protrusion, projected area and aspect ratio were performed with the ImageJ software. Cell protrusion thickness was measured if the protrusion was larger than one pixel in width since the smaller protrusions may not always be visible depending on imaging depth inside the collagen gel under the present imaging conditions. Boyden-chamber cell migration assay MDA-MB-231 cells (510 4 ) or 4T1 Cells (110 5 ) suspended in 100 μl starvation medium were added to the upper chamber of an insert (6.5 mm diameter, 8 μm pore size; Becton Dickson), and the insert was placed in a 24-well plate containing 700 μl starvation medium with or without 10% FBS. When used, inhibitors were added to both the upper and the lower chambers. Migration assays were performed for 6 h and cells were fixed with 3.7% formaldehyde. Cells were stained with crystal violet staining solution, and cells on the upper side of the insert were removed with a cotton swab. Three randomly selected fields (ten objectives) on the lower side of the insert were photographed, and the migrated cells were counted. Migration was expressed as average number of migrated cells in a field. Soft-agar colony formation assays 4T1 cells and MDA-MB-231 cells were maintained in RPMI supplemented with penicillin/streptomycin and 10% FBS. Anchorage-independent cell growth was assessed by the soft agar colony formation assay. Briefly, 2 ml of 0.8% agar was added to each well of a 12-well plate. Detached cells (with or without 150 μM G2) were mixed with an agarose suspension (0.4% final concentration), and then layered onto the 0.8% agarose underlay. Culture medium was changed every 3 days, and the number of cell foci ≥100 mm in diameter was counted after 2 weeks). Each experiment was performed in triplicate. Caspase assay Caspase activity assay was performed as described [60] . Briefly, cells were treated with G2 for different time points. Floating and attached cells (collected by trypsinization) were lysed. Twenty micrograms of cell lysate were then mixed with caspase-3 (Apopain) substrate Rhodamine 110 (AnaSpec; final concentration, 1.5 μM) on ice in a final volume of 20 μl. Samples were then immediately loaded on 96-well plates and fluorescence was measured at 30 °C for 180 min using TECAN at excitation and emission 485 and 535 nm, respectively. Average relative fluorescence units at 120 min were plotted and s.e.m. of at least three independent assays. 4T1 mammary tumour metastasis in mice Female BALB/c mice (6- to 8-week-old) were purchased from Charles River. 4T1 tumour cells (1 × 10 6 ) were injected subcutaneously into the abdominal mammary gland area of mice using 0.1 ml of a single-cell suspension in PBS on day 0. Starting on day 7, when the tumours averaged about ∼ 4–5 mm in diameter, G2 or control solvent were given every day by intraperitoneal injection at 100 mg kg −1 per mouse until day 24. On day 25, the mice were killed. This dosage regiment was well tolerated with no signs of overt toxicity. Every group included five mice. Numbers of metastatic 4T1 cells in lungs were determined by the clonogenic assay. In brief, lungs were removed from each mouse on day 25, finely minced and digested in 5 ml of enzyme cocktail containing 1 × PBS and 1 mg ml −1 collagenase type IV for 2 h at 37 °C on a platform rocker. After incubation, samples were filtered through 70-μm nylon cell strainers and washed twice with PBS. Resulting cells were suspended, plated with a series of dilutions in 10 cm tissue culture dishes in RPMI 1640 medium containing 60 μM thioguanine for clonogenic growth. As 4T1 tumour cells are resistant to 6-thioguanine, metastasized tumour cells formed foci after 7 days, at which time they were fixed with methanol and stained with 0.03% methylene blue for counting. MDA-MB-231 human breast tumour metastasis in mice All animal work was performed in accordance with protocols approved by the Institutional Animal Care and Use Committee of Weill Medical College of Cornell University. Athymic Nude (Foxn1 nu ) immunodeficient mice were purchased from Harlan Laboratory. MDA-MB-231 human breast tumour cells expressing the enhanced GFP-luciferase fusion protein were trypsinized and washed with PBS twice. Mice were anaesthetized with 2% isoflurane. 10 6 cells in 0.1 ml PBS were injected into the lateral tail vein using a 27 × ½’’ gauge needle. The mice were immediately placed onto black pad in the IVIS imaging box and imaged ventrally. Animals were imaged once a week for 7 weeks. G2 was i.p. injected at 100 mg kg −1 daily. Pharmacokinetic study of G2 in mice The pharmacokinetics of G2 were determined in B6D2F1 mice following a single intravenous dose (20 mg per kg body weight). Blood samples were collected into EDTA-coated tubes at time intervals from 5 min to 4 h post dose and centrifuged at 1,500 g for 15 min to generate plasma samples. Pharmacokinetic parameters, including the area under the curve, the peak plasma concentration of G2 after administration ( C max ) and half-life ( T 1/2 ), were estimated from two-compartment fit to the data. Plasma samples were extracted with a mixture of acetonitrile, 0.1% formic acid and water, mixed and centrifuged. The supernatants were analysed using an Agilent HPLC/MS (6120) equipped with a Kinetex C18 (100 × 3 mm 2 , 2.6 μm particle size) column and guard column. Standard curves were prepared by spiking compounds into control plasma, and these were used to determine the drug concentrations. India ink assay To analyse tumour metastasis to the lungs, mice were killed and their lungs were removed and injected with India ink to visualize individual tumour nodules. Briefly, isolated lungs were intra-tracheal injected with India ink (15% India Ink, 85% water, 3 drops NH 4 OH/100 ml). India ink-injected lungs were washed in Feket’s solution (300 ml 70% EtOH, 30 ml 37% formaldehyde, 5 ml glacial acetic acid) and then placed in fresh Feket’s solution overnight. Tumour nodules do not absorb India ink, which results in the normal lung tissue staining black and the tumour nodules remaining white. IVIS imaging For the IVIS system, exposure time is adjusted so that there is no saturated signal. Images are taken using 8 bin at level D. For image acquisition, unit was set to ‘counts’. To quantify the signals, a region of interest was chosen and ‘photons’ was used. In this mode, the measurement or image displays automatically take into account the various settings of integration time, binning, f/stop and field-of-view. Histology Mice were anaesthetized and subsequently perfused with PBS and PBS-buffered 4% paraformaldehyde. Lungs were inflated with 1% low-melting agarose, processed for paraffin-embedded sectioning at 8 μm and stained with H&E. Mouse toxicity study NOD-SCID immunodeficient mice (6- to 8-week-old female mice, n =3 per group) were dosed with either control vehicle (DMSO) or 100 mg kg −1 G2 compound i.p. daily, 5 days per week, for 2 weeks. Body weights and clinical signs were recorded daily. At time of killing (day 15) the mice, blood was collected for clinical chemistry analysis, and complete necropsy was performed on all mice. Tissues were fixed, processed, embedded in paraffin, sectioned and stained with H&E. Major organs, including the heart, lung, kidney, spleen, liver, pancreas, lymph nodes and intestines, were examined microscopically. Statistical analysis Data are expressed as mean±s.e.m. and analysed by Student’s t -test with significance defined as P <0.05. How to cite this article: Huang, F.-K. et al . Targeted inhibition of fascin function blocks tumour invasion and metastatic colonization. Nat. Commun . 6:7465 doi: 10.1038/ncomms8465 (2015).